Reply to ‘Inconclusive evidence for rapid adaptive evolution’ 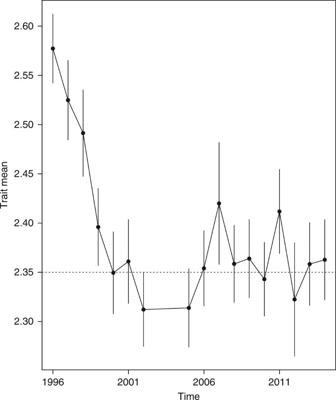Fig. 1 The evolution of log body mass over time, corrected for seasonal variation linked to capture date. We regressed capture date (days away from the center of the breeding season (July 1st)) on log body mass (the dependent variable), having year a factor. Vertical error bars signify one standard error. The data reveal a negative trend in body mass consistent with an OU-model. The dotted line represents the estimated adaptive optimum (θ) for log body mass (2.35) 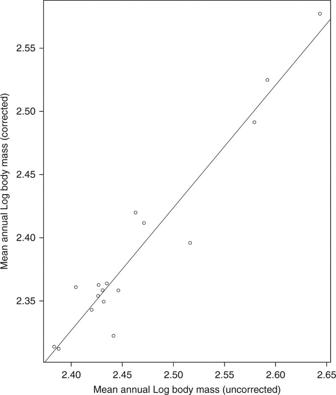Fig. 2 Regression between uncorrected mean annual estimates of Log body mass (from Sætre et al.1) and corrected mean annual estimates of log body mass (the values predicted by the first ANCOVA model, where we regressed capture date (days away from the center of the breeding season (July 1st)) on log body mass (the dependent variable), having year a factor). The data show a strong concordance between both estimates (R2= 0.92;P= 8.29e−10) Statistical analyses We analyzed ANCOVA models where we regressed capture date on log body mass (the dependent variable), having year as a factor. We assumed a common coefficient for how body mass changes as a function of capture date due to the modest sample sizes of measured birds per year. In the first ANCOVA model, capture date was measured as “days away from the center of the breeding season (July 1st)”. We tested the correlation between the annual body mass data used in our original publication and the annual body mass data corrected for seasonal variation with this model, and there is a strong concordance between both estimates ( R 2 = 0.92; P = 8.29e−10, Fig. 2 ). In the second ANCOVA model, capture date was implemented as “days after May 1st” as a quadratic term (with the linear term also included in the model). The third model is a linear mixed-effect model implemented using the lme4 package [10] where log body mass was the dependent variable, year was a fixed effect and month (the month birds where captured) was implemented as a random factor. We note that there are several other non-linear models we could have used, which may have fitted the data better. However, we believe it is best to avoid complex, parameter-rich models given our limited sample size. Fig. 2 Regression between uncorrected mean annual estimates of Log body mass (from Sætre et al. [1] ) and corrected mean annual estimates of log body mass (the values predicted by the first ANCOVA model, where we regressed capture date (days away from the center of the breeding season (July 1st)) on log body mass (the dependent variable), having year a factor). The data show a strong concordance between both estimates ( R 2 = 0.92; P = 8.29e−10) Full size image For each model, we used the predicted mean and variance to compare the goodness of fit of a neutral (unbiased random walk) and an adaptive (OU) model using the PaleoTS package [11] in R. We used bias-corrected AICc as a measure of model fit, and to show the relative support for the two models we used Akaike weights (transformations of the AICc scores to make them sum to one). We also conducted a log-likelihood ratio test using the log-likelihood estimates from the models. Data availability The data are available from the Dryad Digital Repository (doi: 10.5061/dryad.kg3hp51).